Polarization screening-induced magnetic phase gradients at complex oxide interfaces Thin-film oxide heterostructures show great potential for use in spintronic memories, where electronic charge and spin are coupled to transport information. Here we use a La 0.7 Sr 0.3 MnO 3 (LSMO)/PbZr 0.2 Ti 0.8 O 3 (PZT) model system to explore how local variations in electronic and magnetic phases mediate this coupling. We present direct, local measurements of valence, ferroelectric polarization and magnetization, from which we map the phases at the LSMO/PZT interface. We combine these experimental results with electronic structure calculations to elucidate the microscopic interactions governing the interfacial response of this system. We observe a magnetic asymmetry at the LSMO/PZT interface that depends on the local PZT polarization and gives rise to gradients in local magnetic moments; this is associated with a metal–insulator transition at the interface, which results in significantly different charge-transfer screening lengths. This study establishes a framework to understand the fundamental asymmetries of magnetoelectric coupling in oxide heterostructures. Doped La 1− x A x MnO 3 manganese perovskite oxides have received considerable attention for spintronic applications, since they offer many handles for structural control of magnetism and possess a relatively high ferromagnetic (FM) Curie temperature ( T C ≈360 K) [1] , [2] , [3] . In these compounds, A is an alkaline earth such as Ba 2+ , Sr 2+ or Ca 2+ ; for alloying in the range of 0< x <1, the charge state of Mn ions is between the nominal values, 3+ and 4+(ref. 3 ). The electronic configuration for such a 3 d Mn 3+ δ cation in an octahedral crystal field can be written as and , where the magnitude of δ depends on the concentration of x and the degree of hybridization with the neighbouring O 2 p states in the MnO 6 octahedra. In the present work, we focus specifically on the La 1− x Sr x MnO 3 (LSMO) system at compositions near x ≈0.3, where double-exchange interactions dominate, electrons become delocalized, and a completely spin-polarized FM ground state is stabilized [3] . One of the intriguing aspects of the and configurations is the δ -electrons in the e g electronic states. Practically, one may achieve control of electrons by interfacing LSMO with a functional substrate, such as a ferroelectric material like Pb(Zr x Ti 1− x )O 3 (PZT), BaTiO 3 (BTO) or BiFeO 3 (BFO), through controlled growth in a thin-film heterostructure [4] , [5] , [6] . In this class of artificial magnetoelectrics, it has been shown that the magnetic order is coupled with the ferroelectric order at the interface, thereby permitting reversible electric field tuning of T C and transport properties [5] , [7] . The use of a ferroelectric substrate provides several mechanisms to control magnetization, including the screening of bound surface charge from the ferroelectric by metallic carriers in the ferromagnet [4] , [8] , [9] . Poling of the ferroelectric towards or away from the ferromagnet changes the effective charge state at the interface, resulting in a reversible change in local Mn ion valence and spin state [10] , [11] . This charge-transfer screening phenomenon, already widely employed in semiconductor p–n junctions, typically operates over a few unit cells (UCs) and greatly depends on interface structure and chemistry [8] , [12] , [13] . There are many unresolved questions about the nature of this coupling mechanism in the LSMO/PZT system. Pioneering X-ray absorption spectroscopy (XAS) and magneto-optical studies by Vaz et al. [10] found evidence for charge-transfer screening that is estimated to occur over 1–2 UCs at the interface and depends on the PZT polarization direction [11] , [14] , [15] . However, this effect alone was insufficient to explain the measured interface magnetization, so the authors suggested that an associated spin structure change may also occur. We have recently shown that charge-transfer screening acts in concert with local strain fluctuations to mediate coupling, and that the dominant coupling mechanism appears to depend on film geometry [16] . Moreover, it is known that a suppression of ferroelectric polarization may occur at interfaces, but it is unclear how this may play a role in the LSMO/PZT system [17] . Recently, Lu et al. [18] have proposed a theoretical mechanism whereby charge-transfer screening electrostatically dopes an interface region of the LSMO into a paramagnetic insulating state, which might explain the larger screening lengths we and others have measured [16] , [19] . More insight is clearly needed into local ferroelectric polarization and the presence of such a ‘doping-induced double layer,’ which would have fundamental implications for oxide-based electronics. Aberration-corrected scanning transmission electron microscopy (STEM) is an ideal technique to study the local ferroelectric polarization, valence and interfacial electromagnetic phases at spatial regimes inaccessible by traditional surface probes. For instance, Kwon et al. [20] and others have shown that it is possible to relate structure and chemistry measured by STEM to magnetic ion spin state, providing a way to link structure and magnetization at the atomic scale. Here, we directly probe chemistry and valence across the LSMO/PZT/LSMO heterostructure, which we then correlate to measurements of local magnetization, ferroelectric polarization and density functional theory (DFT) calculations. In the present study, we use electron energy loss spectroscopy (EELS) to focus primarily on changes in the O K edge fine structure, which is known to be an indicator of the local electronic configuration of the manganites [21] , [22] , [23] . We combine our experimental EELS results with electronic structure calculations and detailed local measurements of ferroelectric polarization to give direct, spatially resolved insight into spin configurations at oxide interfaces. We find that the local ferroelectric polarization is different at each interface, and that this leads to gradients in the associated magnetic and electronic interfacial phases. This approach serves not only to extend our understanding of the coupling mechanisms in this system, but also informs the broader field of interfacial magnetism. Sample growth We have used a substrate-induced self-poling technique to spontaneously pole the PZT layer during growth, as previously described [16] . We first deposited a ∼ 12nm La 0.7 Sr 0.3 MnO 3 layer onto a bulk SrTiO 3 (001) (STO) substrate using pulsed laser deposition. This method sets the appropriate electrostatic boundary conditions to spontaneously self-pole the PZT ‘up’ or ‘away’ from the STO substrate [16] , [17] , [24] , [25] , [26] , [27] . We then deposited a ∼ 37nm thick PbZr 0.2 Ti 0.8 O 3 layer and a second ∼ 19nm thick LSMO layer. Assuming a uniform, nearly monodomain configuration, this single sample will possess the two different LSMO interface charge states: the top layer will be in a hole charge depletion state and the bottom layer will be in an accumulation state [14] . While dynamic switching of polarization is potentially a more ideal approach to probe these effects, the large-area contacts needed for neutron measurements (several mm 2 ), as well as the difficulty of electrical biasing during EELS, preclude such an experiment. Furthermore, no special care was taken to assure a given termination at these interfaces during growth, and some mixture of termination is expected at each interface, as confirmed by STEM measurements. Finally, we expect little impact from the STO/LSMO and LSMO/Air interfaces, since the LSMO layers are sufficiently thick to isolate PZT interface effects from these interfaces. In the present study, we therefore make no a priori assumptions about interface termination or innate screening; instead we measure a convolution of multiple effects near each interface to develop a holistic understanding of the fundamental asymmetries of magnetoelectric coupling in oxide heterostructures. Electron energy loss spectroscopy EELS linescans were collected from several parts of the film to study the spatial evolution of local Mn valence normal to the PZT interface. In addition to 2D EELS mapping, we employ an enhanced linescan method, termed a ‘SMART’ linescan [28] ; this approach averages a larger area of the interface, reducing the risk of beam damage to the film and increasing the signal-to-noise ratio of the scan, thus ensuring an accurate interpretation of the EELS fine structure. 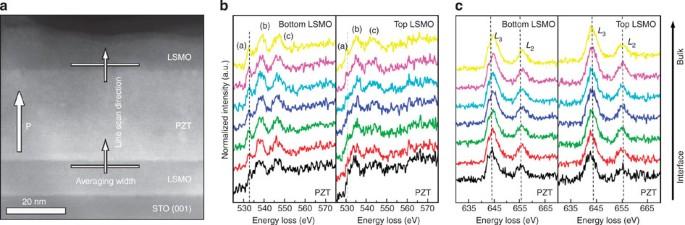Figure 1: Structural and chemical mapping of the heterostructure. (a) Cross-sectional STEM-HAADF micrograph of the film structure, with the direction of ferroelectric polarization and example SMART linescan paths indicated. Separate high-resolution linescans were taken at each interface. The horizontal lines indicate the direction of averaging parallel to the interface. (b) Power-law subtracted EEL spectra corresponding to the OKedge, collected at every lattice plane beginning at the LSMO/PZT interface. (a,b,c) Pre-, main- and secondary-peak features, respectively. (c) Power-law subtracted EEL spectra corresponding to the MnL2,3edge. The rightmost arrow indicates the progression in scans from the PZT interface into the bulk of each LSMO layer. We note that only the first∼10 nm of the top LSMO layer remains after sample thinning. Figure 1a shows an aberration-corrected STEM high-angle annular dark-field (STEM-HAADF) image of the overall heterostructure, in which all the layers are clearly resolved. The top interface exhibits only minimal intermixing across 1–2 atomic planes, while the bottom interface is slightly sharper and exhibits intermixing over just 0–1 atomic plane (see Supplementary Note 1 and Supplementary Figs 1–2 for more details). Spectra for the O K and Mn L 2,3 edges were measured as a function of position normal to the interface and are shown in Fig. 1b,c (the La M 4,5 and Ti L 2,3 edges, also resolved, are not shown here). These scans allow us to measure fine structure changes in both the vicinity of the PZT and the bulk of the LSMO layers. Figure 1: Structural and chemical mapping of the heterostructure. ( a ) Cross-sectional STEM-HAADF micrograph of the film structure, with the direction of ferroelectric polarization and example SMART linescan paths indicated. Separate high-resolution linescans were taken at each interface. The horizontal lines indicate the direction of averaging parallel to the interface. ( b ) Power-law subtracted EEL spectra corresponding to the O K edge, collected at every lattice plane beginning at the LSMO/PZT interface. ( a , b , c ) Pre-, main- and secondary-peak features, respectively. ( c ) Power-law subtracted EEL spectra corresponding to the Mn L 2,3 edge. The rightmost arrow indicates the progression in scans from the PZT interface into the bulk of each LSMO layer. We note that only the first ∼ 10 nm of the top LSMO layer remains after sample thinning. Full size image The O K edge is highly sensitive to the local bonding environment and can be used as an indicator of Mn valence changes [22] , [29] , [30] . This edge, in the dipole approximation, selectively probes the density of unoccupied states of O atoms with 2 p character arising from the first-order transition of electrons from O 1 s to 2 p states. The configuration interaction via hybridization, between the unoccupied states of O 2 p and Mn 3 d symmetry manifests as unique pre-peak spectral signatures, whose weight and peak positions reflect the oxidation state or valence of the Mn cations [22] , [30] , [31] , [32] . Here we probe the O K edge at both the top and bottom LSMO/PZT interfaces to directly map and link the magnitude and direction of ferroelectric polarization to Mn valence state. The O K edge fine structures for the bottom and top interfaces are shown in Fig. 1b , in which both the pre- and main-peak are clearly resolved. We observe three prominent features (labelled a – c ), which correspond to excitations associated with hybridized states of O 2 p states with Mn 3 d , La 5 d /Sr 4 d and Mn 4 sp bands, respectively [22] . We find that the pre- to main-peak energy separation (Δ E O(b−a) ) changes in the vicinity of the LSMO/PZT interface, as shown in Fig. 2a,b . In both cases, the samples display a decrease in separation from a bulk value of ∼ 5.5–6 eV; this decrease is small for the bottom LSMO (see Fig. 2a ), ∼ 0.5 eV over 1 nm, but is nearly double for the top LSMO (see Fig. 2b ), ∼ 1.0 eV over 2.5–3 nm. These energy separations (Δ E O(b−a) ) may be correlated to changes in the Mn valence near the interface [22] ; however, because it is difficult to draw comparisons with absolute valence, we instead focus on the overall trends in behaviour (these trends are further supported by shifts in the O K pre-peak intensity, described in Supplementary Note 2 and Supplementary Fig. 3 ). 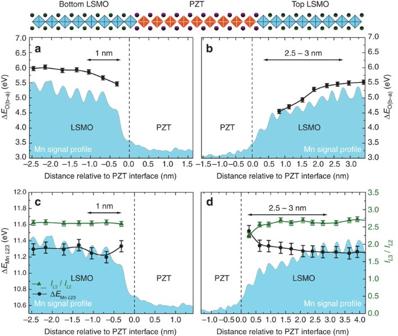Figure 2: EELS measurements of the heterostructure. Local changes in OKedge fine structure are overlaid with an illustration of the heterostructure. (a,b) The OKpre- to main-peak separation (ΔEO(b−a)) in the vicinity of the PZT interface for the bottom and top LSMO layers, respectively. The bottom layer exhibits a small (∼0.5 eV) change, while the top layer exhibits a much larger (∼1 eV) change. The bottom layer shows this change over <1 nm, while the top layer shows a much broader region of change, nearly 2.5–3 nm. (c,d) The difference in MnL2,3edge peak position (black circles) andL3/L2peak intensity ratio (green triangles) in the vicinity of the PZT interface for the bottom and top LSMO layers, respectively. This figure is a combination of separate high-resolution scans at the interface. The edges were fitted using a combination of Gaussian functions in OriginPro and the standard error of each fit was used to calculate the error bars. The difference in bulk energy separations is likely the result of different sample thicknesses on either side of the PZT formed during sample preparation. Figure 2: EELS measurements of the heterostructure. Local changes in O K edge fine structure are overlaid with an illustration of the heterostructure. ( a , b ) The O K pre- to main-peak separation (Δ E O(b−a) ) in the vicinity of the PZT interface for the bottom and top LSMO layers, respectively. The bottom layer exhibits a small ( ∼ 0.5 eV) change, while the top layer exhibits a much larger ( ∼ 1 eV) change. The bottom layer shows this change over <1 nm, while the top layer shows a much broader region of change, nearly 2.5–3 nm. ( c , d ) The difference in Mn L 2,3 edge peak position (black circles) and L 3 / L 2 peak intensity ratio (green triangles) in the vicinity of the PZT interface for the bottom and top LSMO layers, respectively. This figure is a combination of separate high-resolution scans at the interface. The edges were fitted using a combination of Gaussian functions in OriginPro and the standard error of each fit was used to calculate the error bars. The difference in bulk energy separations is likely the result of different sample thicknesses on either side of the PZT formed during sample preparation. Full size image We have also studied changes in the Mn L 2,3 edge, which is associated with excitations from the spin-orbit split 2 p 3/2 and 2 p 1/2 levels to available states in the 3 d band [22] , [33] . We focus on the chemical shift of the Mn L 2,3 edge, which only depends on core-level energy and the effective charge of the atom [34] . This method directly measures atomic charge, independent of background subtraction and sample thickness [29] . Figure 1c shows the Mn L 2,3 edge fine structures for both the bottom and top LSMO layers. Taking the dashed lines as a guide to the eye, there is a clear shift to lower energy in the vicinity of the PZT interface, indicating the local chemical state changes. Fig 2c,d shows that in both cases the edge intensity ratio remains nearly constant throughout the LSMO. However, the Mn L 2,3 edge separation displays very different behaviour for the two interfaces. In both cases, the samples display a bulk value of ∼ 11.2–11.3 eV that deviates in the vicinity of the PZT interface; the bottom LSMO (see Fig. 2c ) displays a slight fluctuation of ∼ 0.1 eV over 1 nm, while the top LSMO (see Fig. 2d ) displays a steady increase of nearly ∼ 0.2–0.3 eV over a broad 2.5–3nm region. The spatial extent of these regions in particular agrees well with the trends observed in the O K edge energy separation (see Fig. 2a,b ). Density functional theory To probe the structural and chemical origin of these EELS features, as well as their relationship with local phases, we have conducted DFT+ U calculations using the planewave pseudopotential method as implemented in the Quantum Espresso package [35] ; the O K edge X-ray absorption spectra were calculated with the help of the XSpectra package [36] , [37] . We note that although EELS and XAS are not, strictly speaking, equivalent, these spectroscopy techniques probe the same electronic states: comparisons of experimental and theoretical spectra across the two techniques thus provide invaluable insight and are commonly used to rationalize observed trends and fine structure features. Moreover, in our O K edge spectra calculations, we set the X-ray momentum and X-ray polarization vectors to be the same. Within the dipole approximation, when the X-ray momentum vector and X-ray polarization vectors are equal, the EEL spectrum is directly equivalent to the X-ray absorption cross-section (see ref. 38 ). The core and valence electrons were treated with ultrasoft pseudopotentials [39] and the PBEsol exchange-correlation functional [40] . We apply the plus Hubbard- U correction within the Dudarev formalism [41] using U eff =2 eV (refs 16 , 42 ) to treat the Mn 3 d orbitals (see Methods section for additional calculation details and Supplementary Note 3 and Supplementary Fig. 4 , where we show that trends in O K edge EELS do not change with the choice of U eff ). We consider three unique chemical compositions, La 0.6 Sr 0.4 MnO 3 , La 0.7 Sr 0.3 MnO 3 and La 0.8 Sr 0.2 MnO 3 , permitting us to explore the electronic structure trends for a broad range of chemical doping. In the ground state, all the compositions have a rhombohedral crystal structure (space group ), but they differ in the magnitude of octahedral rotations [43] , [44] , [45] , [46] . From the La 1− x Sr x MnO 3 phase diagram [47] , the three compositions are also expected to be FM and metallic. We note that the ‘nominal’ charge state of Mn is expected to be different in the three compositions, which we confirmed from the calculated magnetic moments (see Supplementary Table 1 ). Our main goal is to disentangle the effect of Mn valence, magnetic spin order, Mn–O–Mn bond distortions, and octahedral rotations on the O K edge spectral features. The La and Sr partial occupancies were simulated by following an approach adapted by Burton et al [48] , [49] . We construct an effective pseudopotential for a ‘fictitious’ atom, whose cutoff radii and valence electron configuration are assumed to be that of a La atom, but whose valence charge is modified to mimic the valence of La/Sr partial site occupancy. For example, in our simulation for La 0.7 Sr 0.3 MnO 3 , the valence charge for the La/Sr atom was taken to be equal to 2.7 + . Because of the constraints placed on the La/Sr partial occupancy, we neither relaxed the internal atomic coordinates nor the UC parameters: instead, we considered the bulk experimental structures and calculated their charge density. Near the LSMO/PZT interface, the Mn–O–Mn bond distortions can be quite different from that in the bulk. We performed additional simulations to assess the response of the O K edge to these distortions. We built a 30-atom supercell (a representation of the primitive 5-atom UC) reflective of La 2/3 Sr 1/3 MnO 3 superlattice and applied an epitaxial strain using the in-plane lattice constant of SrTiO 3 (3.905 Å). We allowed the out-of-plane axis to relax, until the z axis cell pressure became negligibly small and Hellman–Feynman forces became <2 meV Å −1 . Our 30-atom superlattice contains two types of Mn sites: (i) one of the Mn sites is interleaved between the two positively charged [LaO] 1+ planes, where the Mn–O–Mn bond angle is ∼ 180° and (ii) the other Mn site is interleaved between positively charged [LaO] 1+ and neutral [SrO] 0+ planes, where the Mn–O–Mn bond angle is 172.4°, suggesting off-centring of the Mn cation. This off-centring mimics the interfacial Mn–O bond distortions seen in our STEM images, which we discuss later; however, the exact Mn–O–Mn bond angle could not be determined from our STEM images. We then created a 2 × 1 × 1 supercell (with 60 atoms) and calculated the O K edge EELS along the [110] X-ray polarization and momentum vector directions. As a result, our DFT calculations do not directly simulate the complex LSMO/PZT/LSMO heterostructure. Instead, we perform systematic calculations on the bulk structures and superlattices to uncover trends in the O K edge spectra that we may qualitatively correlate to our experimental O K edge EEL spectra. In Fig. 3a–c , we show the total (spin up+spin down) XAS spectra for the FM spin order for the three chemical compositions. 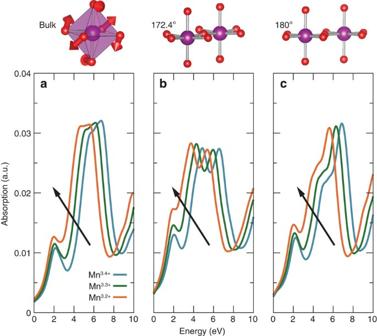Figure 3: Total OKedge spectra calculated from DFT for different distortions. The three curves correspond to three different La1−xSrxMnO3(LSMO) compositions, wherex=0.6 (blue), 0.7 (green) and 0.8 (orange), with the arrow indicating the decrease in valence. (a) The OKedge spectra for the bulk LSMO system with anti-ferrodistortive distortions. Here all the six Mn–O bond lengths are equidistant (1.954 Å). The X-ray polarization and momentum vectors were set along the [100] direction. (b,c) The OKedge of LSMO grown epitaxially on SrTiO3substrate. The X-ray polarization and momentum vectors were set along the [110] direction. We note that inb, the Mn atom is off-centred, which leads to a Mn–O–Mn bond angle of 172.4°. The four equatorial Mn–Oeqbond lengths are 1.957 Å and the two inequivalent apical Mn–Oapbond lengths are 1.904 and 1.960 Å. On the other hand, incthere is no cation off-centring, but the LSMO film is under the influence of tensile epitaxial strain. The four equatorial Mn–Oeqbond lengths are 1.953 Å and the two equivalent apical Mn–Oapbond lengths are 1.9034 Å. Figure 3: Total O K edge spectra calculated from DFT for different distortions. The three curves correspond to three different La 1− x Sr x MnO 3 (LSMO) compositions, where x =0.6 (blue), 0.7 (green) and 0.8 (orange), with the arrow indicating the decrease in valence. ( a ) The O K edge spectra for the bulk LSMO system with anti-ferrodistortive distortions. Here all the six Mn–O bond lengths are equidistant (1.954 Å). The X-ray polarization and momentum vectors were set along the [100] direction. ( b , c ) The O K edge of LSMO grown epitaxially on SrTiO 3 substrate. The X-ray polarization and momentum vectors were set along the [110] direction. We note that in b , the Mn atom is off-centred, which leads to a Mn–O–Mn bond angle of 172.4°. The four equatorial Mn–O eq bond lengths are 1.957 Å and the two inequivalent apical Mn–O ap bond lengths are 1.904 and 1.960 Å. On the other hand, in c there is no cation off-centring, but the LSMO film is under the influence of tensile epitaxial strain. The four equatorial Mn–O eq bond lengths are 1.953 Å and the two equivalent apical Mn–O ap bond lengths are 1.9034 Å. Full size image We find excellent agreement between the experimental (see Fig. 1b ) and our calculated O K edge spectra; specifically the three features (marked as a,b and c) in Fig. 1b are well reproduced in our calculated spectra. For the remainder of the present work, we will focus mainly on the pre- and main-peaks. We find that as the Mn ‘nominal’ valence increases, the spectral weight of the pre-peak feature (corresponding to the O 2 p –Mn 3 d hybridized orbitals) decreases and shifts slightly to higher energies. Despite the differences in the spectral signatures as a result of changes to the Mn–O bond distortions, such as peak splitting and redistribution of spectral weights, the overall Δ E trend as a function of Mn valence remains the same. The main-peak (O 2 p –La 5 d hybridized orbitals), on the other hand, shifts to a higher energy with increasing Mn ‘nominal’ valence. We identify two key features: namely, that the spectral weight of the pre-peak and the energy difference between the pre- and main-peaks are indicators of changes in the Mn valence state in the O K edge. We next repeated the calculations on bulk structures; however, this time we imposed anti-FM- A (AF- A ) spin order on the Mn atoms. We show only the results for the pre-peak spectral features in Fig. 4a , since the main-peak spectral features show little variation between the FM and AF- A spin orders. 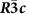Figure 4: Total OKedge spectra calculated from DFT for therhombohedral structure. (a) Comparison of the spectral weight and energies of the pre-peak feature (O 2p–Mn 3dhybridized orbitals) between FM (continuous line) and AF-A(dotted line) spin configurations on the Mn atom for the three compositions. For the AF-Acompositions, the spectral weight increases and the pre-peak shifts to a lower energy, relative to the FM compositions. (b) Pre- and main-peak spectral features for the three bulk structures (FM spin order), where we constrain the valence charge of the La/Sr site to be nominally 2.7+so that the chemical composition of the bulk perovskite compound is fixed at La0.7Sr0.3MnO3for the three structures. We note that in this simulation the rotation amplitudes for the MnO6octahedra are varied. The effect on the EEL spectra is negligible in this case. (c) Calculated energy difference (ΔEin eV) between the pre-and the main-peaks fromFig. 3andbshown as circles and triangles, respectively. (d) Calculated ΔEfor different Mn octahedra rotation amplitudes fromb, showing a negligible change. Figure 4: Total O K edge spectra calculated from DFT for the rhombohedral structure. ( a ) Comparison of the spectral weight and energies of the pre-peak feature (O 2 p –Mn 3 d hybridized orbitals) between FM (continuous line) and AF- A (dotted line) spin configurations on the Mn atom for the three compositions. For the AF -A compositions, the spectral weight increases and the pre-peak shifts to a lower energy, relative to the FM compositions. ( b ) Pre- and main-peak spectral features for the three bulk structures (FM spin order), where we constrain the valence charge of the La/Sr site to be nominally 2.7 + so that the chemical composition of the bulk perovskite compound is fixed at La 0.7 Sr 0.3 MnO 3 for the three structures. We note that in this simulation the rotation amplitudes for the MnO 6 octahedra are varied. The effect on the EEL spectra is negligible in this case. ( c ) Calculated energy difference (Δ E in eV) between the pre-and the main-peaks from Fig. 3 and b shown as circles and triangles, respectively. ( d ) Calculated Δ E for different Mn octahedra rotation amplitudes from b , showing a negligible change. Full size image We find two critical signatures in the pre-peak that differentiate FM from AF- A spin orders: as a general trend, we find that AF- A spin order increases the spectral weight of the pre-peak features and also shifts the pre-peak towards lower energies relative to their FM counterparts. Our DFT calculations corroborate the hypothesis that we can use the pre-peak spectral feature from O K edge measurements to probe the local variation in the Mn valence and the magnetic configurations. This is an important finding, because earlier works on LSMO magnetoelectric heterostructures have shown an AF spin order near the interface arising from the magnitude and direction of ferroelectric polarization [10] , [14] . However, it has been challenging to experimentally probe the spin alignment of Mn atoms near the interface. Our DFT calculations indicate that layer (depth)-resolved O K edge EELS measurements may offer insights to capture the unique spin behaviour of LSMO films. In addition to the two spin configurations, we also probed the effect of octahedral rotations on the O K edge spectral features. Our calculations involved taking the three bulk structures, but we constrained the valence charge of the La/Sr site to be nominally 2.7 + . This fixes the chemical composition of the bulk perovskite compound at La 0.7 Sr 0.3 MnO 3 for the three structures, but allows for different octahedral rotation amplitudes. The resulting O K edge spectra for the FM spin order are shown in Fig. 4b . We find that the octahedral rotations (within the constraints imposed in our calculations) have little effect on the O K edge spectra. In Fig. 4c,d we quantify, from the DFT calculations, the energy difference between the pre- and main-peak spectral features for the FM spin configuration. It is clear that the Mn valence has a dominating influence in determining the energy levels of the hybridized orbitals relative to octahedral or Mn–O–Mn bond distortions. Interfacial phase mapping We now interpret our experimental EELS measurements of the O K edge fine structure to estimate the local phases present at the LSMO/PZT interface. We first compare our measured O K pre- to main-peak energy separation (Δ E O(b−a) ) with our DFT calculations and standards investigated by Varela et al. [22] , as we have already shown in Fig. 2a,b . Far from the interface, we find that the LSMO is in a bulk-like state, with a nominal Mn valence corresponding to the expected La 0.7 Sr 0.3 MnO 3 (Mn ∼ 3.3+ ) doping. We have confirmed this nominal doping using angle-resolved X-ray photoelectron spectroscopy (as described in Supplementary Note 4 and Supplementary Fig. 5 ). We are then able to calculate the effective change in Mn doping relative to this bulk-like state, which we plot as a function of position in Fig. 5a,b . Finally, by comparing this doping evolution with the bulk LSMO phase diagram at room temperature, we are able to estimate the local electronic and magnetic phases present in the vicinity of the PZT interface. 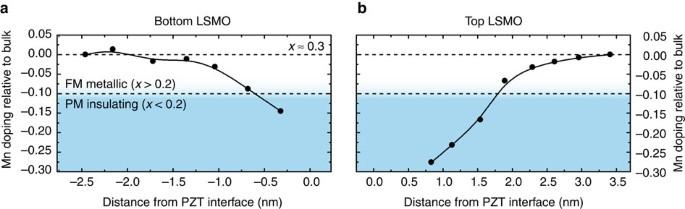Figure 5: Interfacial map of relative Mn valence. Map of local Mn doping relative to bulk La0.7Sr0.3MnO3as a function of position normal to the LSMO/PZT interface for the bottom (a) and top (b) LSMO layers. The boundaries of the associated magnetic and electronic phases are overlaid and estimated from the bulk LSMO phase diagram47. Figure 5: Interfacial map of relative Mn valence. Map of local Mn doping relative to bulk La 0.7 Sr 0.3 MnO 3 as a function of position normal to the LSMO/PZT interface for the bottom ( a ) and top ( b ) LSMO layers. The boundaries of the associated magnetic and electronic phases are overlaid and estimated from the bulk LSMO phase diagram [47] . Full size image Our analysis shows that for the bottom LSMO layer (see Fig. 5a ), the effective Mn doping retains its bulk value up to approximately three lattice planes from the interface, where it drops by ∼ 0.15 over a nanometre. In contrast, the top LSMO layer (see Fig. 5b ) shows a larger ∼ 0.26 drop over a broad 2.5–3nm region. This measurement reveals a clear spatial asymmetry about the PZT layer: the top layer displays a wide region of valence shift, while the bottom layer displays a more narrow region. Furthermore, a comparison of these values with the bulk phase diagram at room temperature shows that the bottom LSMO is almost uniformly FM and metallic, while the top LSMO should be broadly paramagnetic and insulating at the interface [47] . We note that previous studies have found evidence to support the formation of an AF phase at low temperature [10] , [14] . However, at room temperature the transition to a paramagnetic, insulating phase has previously been invoked to explain the anomalously large screening lengths observed in LSMO/BTO and may be responsible for the similarly large lengths we observe here [18] . Interestingly, while a decrease in valence is expected for the top LSMO (depletion state), an increase in valence is actually expected for the bottom LSMO (accumulation state) [14] . However, we find that both interfacial valences decrease near the PZT interface, although the magnitude of the drop for the top LSMO is much larger. The valence decrease of the bottom LSMO may arise from depolarization of the PZT interface, incomplete charge screening and/or intermixing [26] , [50] . Polarized neutron reflectometry Our EELS and DFT results have raised the interesting possibility of spatial gradients in the magnetic and electronic phases at the LSMO/PZT interface. Intuitively, one would expect that the transition from FM metallic to paramagnetic insulating phases at the top LSMO interface would significantly reduce room temperature magnetization. To probe this, we use polarized neutron reflectometry (PNR), a scattering technique that allows us to measure the depth-resolved magnetic structure and is used to isolate individual magnetic layers in a thin-film heterostructure [16] , [51] , [52] , [53] , [54] . 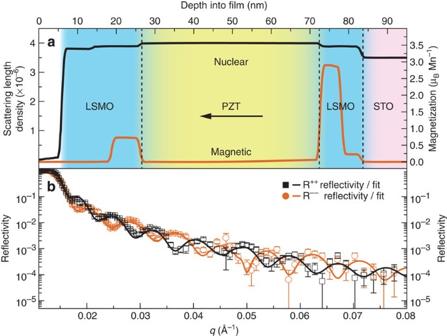Figure 6: PNR measurements of local magnetization. (a) The resulting nuclear scattering length densities (black) obtained from the fit to the data and the associated estimated magnetization (orange). We note some change in nuclear scattering length density near the surface, as well as a reduced magnetization at the STO interface. The arrow indicates the direction of ferroelectric polarization. (b) The measured non-spin-flip reflectivities (shapes), overlaid with a fit to the data (lines). These measurements were conducted at 298 K, with a 1 T field applied along the substrate [100] direction in the plane of the film. Figure 6 shows the result of PNR measurements conducted at 298 K with a 1T field applied along the substrate [100] direction. These measurements were performed on the Magnetism Reflectometer at the Spallation Neutron Source, Oak Ridge National Laboratory [55] . Figure 6b shows the measured non-spin-flip reflectivity, which indicates clear spin splitting resulting from the magnetization of the sample. The calculated fit is overlaid on the data and the resulting scattering length density depth profiles are shown in Fig. 6a . The depth profile reveals that the magnetization of the two LSMO layers is strongly asymmetric: the top LSMO displays a greatly suppressed magnetization throughout , while the bottom LSMO displays a large magnetization that is only reduced at the STO interface. As described in Supplementary Note 5 and Supplementary Fig. 6 , our best-fitted models all point towards the existence of this asymmetry and graded magnetization. We have previously shown that the broad suppression of magnetization near the vacuum surface can result from strain fluctuations; however, at the interface the charge-transfer screening effect largely controls the magnetization [16] . Our results suggest a uniformly FM character for the bottom interface, in agreement with the phase map in Fig. 5a . In contrast, the top LSMO layer possesses a strongly suppressed magnetization near the interface, where strain fluctuations are expected to be minimal, as shown in Fig. 5b [16] . This further supports the idea of magnetic and electronic phase transitions at the interface, in agreement with our EELS and DFT results. Figure 6: PNR measurements of local magnetization. ( a ) The resulting nuclear scattering length densities (black) obtained from the fit to the data and the associated estimated magnetization (orange). We note some change in nuclear scattering length density near the surface, as well as a reduced magnetization at the STO interface. The arrow indicates the direction of ferroelectric polarization. ( b ) The measured non-spin-flip reflectivities (shapes), overlaid with a fit to the data (lines). These measurements were conducted at 298 K, with a 1 T field applied along the substrate [100] direction in the plane of the film. Full size image Polarization screening effects on valence The valence and magnetic changes described in the previous section are the result of a complex interplay of phenomena, including interfacial charge-transfer screening and possible electronic phase transitions [16] , [18] , [56] . As already mentioned, the local screening of bound surface charge is expected to significantly affect Mn ion valence, as well as the formation of interfacial phases; thus, it is important to understand the local ferroelectric polarization at both LSMO/PZT interfaces. Conventional scanning probe techniques, such as piezoresponse force microscopy, are confined to surfaces and are generally of limited use in studying interfaces [57] . However, using aberration-corrected STEM-HAADF, it is possible to directly measure cation displacements with picometre precision, allowing us to characterize local ferroelectric polarization at each LSMO/PZT interface (see Supplementary Note 6 and Supplementary Fig. 7 for details). These results, shown in Fig. 7 , reveal different polarization behaviour for each LSMO/PZT interface. At the bottom interface (see Fig. 7c,d ), the PZT polarization P S ≈53±15 μC cm −2 is nominally constant over the interface region. However, the top LSMO interface (see Fig. 7a,b ) behaviour is markedly different: the average PZT polarization P S ≈70±15 μC cm −2 is >30% larger than the bottom; moreover, within the interface region the polarization is reduced, likely due to incomplete charge screening and/or intermixing with the LSMO. Yu et al. have found that a combination of depolarizing fields and electrostatic differences at asymmetric interfaces can give rise to a preferred orientation of the ferroelectric polarization at each interface [26] . The magnitude of the top polarization agrees well with previous displacement current measurements ( P S ≈85 μC cm −2 ) [14] , but our local measurements show that this polarization can be quite different for each interface. 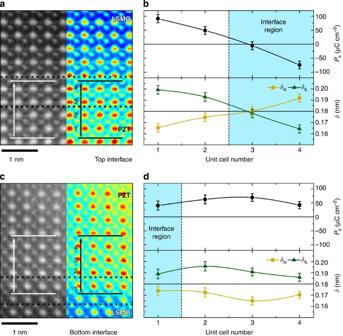Figure 7: STEM-HAADF measurements of local ferroelectric polarization. (a,c) STEM-HAADF greyscale and colorized images for the top and bottom interfaces, respectively. The dashed lines indicate the interface region and the numbers mark the position of the measured unit cells. (b,d) The long (δIL) and short (δIS) Ti4+cation displacement directions, as well as the calculated spontaneous polarization (PS) for the top and bottom interfaces, respectively. These displacements are the result of averaging over several positions parallel to the interface. Figure 7: STEM-HAADF measurements of local ferroelectric polarization. ( a , c ) STEM-HAADF greyscale and colorized images for the top and bottom interfaces, respectively. The dashed lines indicate the interface region and the numbers mark the position of the measured unit cells. ( b , d ) The long ( δ IL ) and short ( δ IS ) Ti 4+ cation displacement directions, as well as the calculated spontaneous polarization ( P S ) for the top and bottom interfaces, respectively. These displacements are the result of averaging over several positions parallel to the interface. Full size image We may estimate the effective bulk alloying change induced by charge-transfer screening, assuming that the polarization is nominally constant parallel to the interface and fully screened by free carriers in the LSMO across a 2–3 UCs ( ∼ 1.2 nm) screening length. On the basis of calculations by Lu et al. [18] , we may estimate Δ x = P S × a , where a ≈0.0041, cm 2 μC −1 . For P S,top ≈70±15 μC cm −2 then, we find Δ x ≈0.29±0.06, while for P S,bottom ≈53±15 μC cm −2 , we find Δ x ≈0.22±0.06. This suggests that the magnitude, as well as the direction, of the screening effect will be different for the top and bottom interfaces. A comparison of this calculation with our EELS phase map shows a striking agreement between the magnitude of bulk valence change (see Fig. 5b ). Our calculation further supports the idea of a transition from FM and metallic to paramagnetic and insulating at this interface at room temperature. The magnitude of the change for the bottom interface is also reduced in both our calculation and our EELS phase map (see Fig. 5a ), but the sign of this change is not fully consistent with the charge-transfer screening model. There has been considerable debate as to the spatial extent of this screening, since calculations of the Thomas–Fermi screening length vary [14] , [15] , [16] , [18] , [58] , [59] , [60] . In the present study, we find that the Mn valence change for the top interface occurs over a broader region than is expected from pure charge-transfer screening (<1.9 nm) [58] , [60] . Lu et al. [18] have proposed a qualitative model for LSMO/BTO that may begin to reconcile both the discrepancies in screening length as well as the interface phase transitions we observe. The authors describe piezoresponse force microscopy measurements of polarization screening, which yield a large ∼ 3nm screening length. They propose that local screening of surface charge acts to push an interface layer of La 0.7 Sr 0.3 MnO 3 into the paramagnetic insulating region of the phase diagram at room temperature, increasing the effective hole doping, and thereby expanding the screening region. Our EELS results (see Fig. 5 ) show that the measured effect on valence is more than sufficient to push the top interface region into the paramagnetic insulating phase at room temperature. Because charge must be screened over this insulating region, the effective screening length is increased. In contrast, the bottom interface is expected to be almost uniformly FM and metallic at room temperature, with an associated short screening length. This is supported by our local measurements of ferroelectric polarization, which show that the magnitude of the bound surface charge at the top interface is adequate to induce such a change, while an ∼ 30% smaller effect is expected for the bottom interface. This mechanism accounts for the behaviour we have observed in our EELS results and is supported by electronic structure calculations, as well as by the asymmetric magnetization behaviour revealed by PNR. Using local probes, we are able to attain direct insight into these features for the first time and we are able to resolve the associated electronic and magnetic phases with unprecedented atomic-scale resolution. Our results begin to unravel the connections between charge, valence and spin configurations in these materials. Using EELS, we are able to quantify the extent of charge-transfer screening effects and we show that they depend on the polarization direction. We directly measure the local Mn valence and associated O K edge fine structure changes to construct a map of interfacial phases. Our DFT calculations lend support to the presence of asymmetric magnetic phase transitions, as reflected in EELS fine structure changes, which we are able to qualitatively reproduce. Our STEM-HAADF measurements of local atomic displacements reveal that the local ferroelectric polarization at the top interface is nearly 30% larger than the bottom interface and is large enough to induce a transition deep into an insulating, paramagnetic phase at the LSMO interface at room temperature. We combine these local chemical analyses with PNR measurements, which reveal a strongly asymmetric magnetic ordering about the PZT layer, likely originating from charge-transfer screening. There may also be additional contributions from differing terminations and defect formation at the two interfaces, as has been previously observed in BTO/LSMO [61] and BFO/LSMO [62] . However, in the present study, we describe the overall behaviour of the system, focusing on the major factors controlling this behaviour, and we have not attempted to isolate every mechanism at work. Collectively, these results suggest a magnetic phase transition at the LSMO/PZT interface, in agreement with other studies [14] , [63] , [64] . We find that the local ferroelectric polarization differs at each interface, which affects the magnitude of the charge-transfer screening effect in each LSMO layer. Our results suggest a large change in Mn valence at the top LSMO interface, which gives rise to the suppression in magnetization that we measure in PNR. We believe that the functionality of devices based on similar heterostructures will be greatly affected by intrinsic spontaneous polarization of the chosen ferroelectric. For instance, for Pb(Zr 0.55 Ti 0.45 )O 3 , P S ≈70–85 μC cm −2 , while for BTO and BFO, P S ≈48 μC cm −2 and P S ≈50–60 μC cm −2 , respectively [14] , [18] , [65] . Any suppression or enhancement of ferroelectric polarization will be even more pronounced in the latter compounds. It may be possible to tune the boundary region with polarization by further reducing the hole doping of the system, which may be achieved by increasing Sr doping, at the cost of reducing T C from its maximum in La 0.7 Sr 0.3 MnO 3 . Further study into the polarization- and composition-dependent phase diagram is needed; the stacking sequence of the layers in the heterostructure may also play a critical role in device performance. Regardless, it is clear that models of magnetoelectric coupling in the manganites and related systems must begin to account for interfacial phase transitions, which may drastically alter coupling behaviour. Thin-film growth PbZr 0.2 Ti 0.8 O 3 films were grown by pulsed laser deposition at 635 °C at 100 and 200 mTorr pO 2 , with laser repetition rates of 12 and 3 Hz, and laser fluences of 1.75 and 2 J cm −2 , respectively. The La 0.7 Sr 0.3 MnO 3 layers were grown at 650 °C at 200 mTorr of oxygen with a laser repetition rate of 2 Hz and a fluence of 1.5 J cm −2 . Films were then cooled to room temperature in 760 Torr pO 2 . Transmission electron microscopy Samples were prepared for TEM by conventional mechanical polishing and ion milling. HRTEM images were captured at 200 keV on a JEOL 2100 LaB 6 . EELS maps and STEM-HAADF images were collected on a C S -corrected Nion UltraSTEM 100 operating at 100 keV, with a convergence angle of 30 mrad and an effective energy resolution of 0.4–0.7 eV (depending on the energy dispersion used: a higher dispersion was chosen for improved precision on the energy shift measurements, specifically for the O K and Mn L 2,3 fine structure analysis, while lower dispersions allowed for detection of the largest possible range of edges for overall chemical profiling of the films) [66] . The background was removed from each scan using a power-law fit. The spectra were offset to the known onset of the O K edge. To improve the signal-to-noise ratio of the STEM-HAADF data while minimizing sample damage, a high-speed time series was recorded (5 μs per pixel). This data set was first rigid registered to eliminate any sample or stage drift (L. Jones et al., Smart Align - A New Tool for Robust Rigid Non-Rigid Registration of Scanning Microscope Data (Submitted to Adv. Struct. Chem. Imaging)). High-frequency scan-noise was then compensated using the Jitterbug software (available from HREM Research at http://www.hremresearch.com ). Importantly, the scan-noise was compensated in each individual frame of the series before averaging across the series [67] . The data were not smoothed or filtered in any way. Measurements of local ferroelectric polarization are described in Supplementary Note 6 . Density functional theory In our DFT calculations, we explored both FM and A -type AF spin configurations. In AF spin order, the in-plane Mn atoms are ferromagnetically aligned, whereas the out-of-plane Mn atoms are antiferromagnetically coupled with one another. Semicore 3 s and 3 p states were included in the valence electron configuration for the Mn atom (for La, Mn and O atoms, we used the valence electron configuration of 5 s 2 5 p 6 6 s 2 5 d 1 , 3 s 2 3 p 6 3 d 5 4 s 2 and 2 s 2 2 p 4 , respectively). We used a 90 Ry plane-wave cutoff for the wavefunctions and a 900 Ry cutoff for the kinetic energy, an effective Hubbard- U value of 2 eV to treat the correlated Mn 3 d electrons, the Marzari–Vanderbilt smearing method [68] with a width of 0.02 Ry, a 4 × 6 × 4 (for the bulk structure) and 4 × 4 × 4 (for the superlattice) k -grid [69] centred at Γ for the self-consistent field (SCF) calculation, a 10 −8 eV convergence threshold for the total energy in the SCF calculation, and a 4 × 4 × 2 mesh with 64 total (spin up+spin down) k -points in the irreducible Brillouin zone for the O K edge EELS calculation. We introduced a core-hole into the O-pseudopotential of the absorbing atom, which we compensated in our SCF calculation by adding a background charge of +1 e . Additional calculation details for the O K edge spectra include: a 0.5 eV broadening parameter and a 10 −5 eV convergence threshold for the Lanczos method. Polarized neutron reflectometry PNR was conducted at 298 K with an in-plane magnetic field of 1 T applied along the [100] substrate direction on the Magnetism Reflectometer at the Spallation Neutron Source, Oak Ridge National Laboratory. Non-spin-flip specular reflectivites were measured from q =0.005–0.1 Å −1 . The reflectivity data were then fit with the ReflPak software package [70] and refined in conjunction with X-ray diffraction data. A fit was conducted with uniform magnetization in the LSMO layers and a second fit was conducted in which the magnetization was allowed to vary. It was found that the some variation in the chemical scattering length density near the surface was needed to fit the data most accurately. How to cite this article : Spurgeon, S. R. et al. Polarization Screening-Induced Magnetic Phase Gradients at Complex Oxide Interfaces. Nat. Commun. 6:6735 doi: 10.1038/ncomms7735 (2015).